Doping of polycrystalline CdTe for high-efficiency solar cells on flexible metal foil Roll-to-roll manufacturing of CdTe solar cells on flexible metal foil substrates is one of the most attractive options for low-cost photovoltaic module production. However, various efforts to grow CdTe solar cells on metal foil have resulted in low efficiencies. This is caused by the fact that the conventional device structure must be inverted, which imposes severe restrictions on device processing and consequently limits the electronic quality of the CdTe layer. Here we introduce an innovative concept for the controlled doping of the CdTe layer in the inverted device structure by means of evaporation of sub-monolayer amounts of Cu and subsequent annealing, which enables breakthrough efficiencies up to 13.6%. For the first time, CdTe solar cells on metal foil exceed the 10% efficiency threshold for industrialization. The controlled doping of CdTe with Cu leads to increased hole density, enhanced carrier lifetime and improved carrier collection in the solar cell. Our results offer new research directions for solving persistent challenges of CdTe photovoltaics. Emerging photovoltaic (PV) technologies based on thin films of Cu(In,Ga)Se 2 (refs 1 , 2 ), Cu 2 ZnSn(S,Se) 4 (ref. 3 ), CdTe [4] , [5] or silicon [6] , as well as dye-sensitized [7] and organic materials [8] have the potential to significantly reduce the cost of solar electricity. CdTe-based PV offers the shortest energy payback time among all PV technologies [9] and has the second largest market share after the conventional crystalline silicon technology. Its energy return on investment exceeds that of oil-fired electricity [10] and its compliance with environmental and safety standards is demonstrated by several studies [11] . 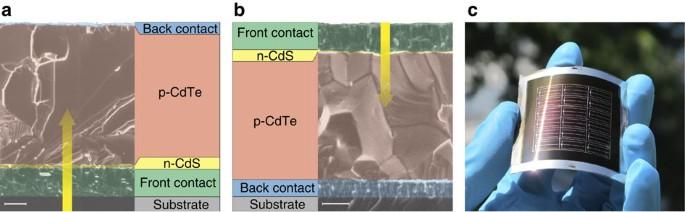Figure 1: CdTe solar cells. (a,b) Scanning electron micrograph and schematic of the cross-section of a CdTe solar cell in the conventional superstrate configuration (a) and the substrate configuration (b) which allows the use of opaque substrates like metal foils. In substrate configuration Mo/MoOxand i-ZnO/ZnO:Al are used as electrical back and front contact, respectively. The scale bars correspond to 1 μm. The yellow arrows show the direction of illumination. (c) Photograph of a sample with several CdTe solar cells on flexible metal foil. Figure 1a shows the cross-section of the conventional CdTe solar cell structure, which has been mainly followed over the past 40 years [4] , [12] . In this ‘superstrate configuration’, light enters through the substrate into the solar cell, limiting the choice of substrates to transparent materials. In contrast to that, the inverted structure or ‘substrate configuration’ ( Fig. 1b ) allows the use of flexible metal foil substrates ( Fig. 1c ), which is expected to lead to a significant price reduction of CdTe PV by implementing high-throughput roll-to-roll manufacturing. However, solar cells in substrate configuration have previously exhibited considerably lower efficiencies than in superstrate configuration, with the highest published efficiency of CdTe solar cells on metal foil remaining below 8% (refs 13 , 14 , 15 , 16 , 17 , 18 ). Figure 1: CdTe solar cells. ( a , b ) Scanning electron micrograph and schematic of the cross-section of a CdTe solar cell in the conventional superstrate configuration ( a ) and the substrate configuration ( b ) which allows the use of opaque substrates like metal foils. In substrate configuration Mo/MoO x and i-ZnO/ZnO:Al are used as electrical back and front contact, respectively. The scale bars correspond to 1 μm. The yellow arrows show the direction of illumination. ( c ) Photograph of a sample with several CdTe solar cells on flexible metal foil. Full size image One of the major challenges of CdTe solar cell research is the achievement of a high hole density in the CdTe layer by means of controlled acceptor doping. It is impeded by the spontaneous formation of compensating donors, a phenomenon commonly observed in the field of II–VI semiconductors [19] . For example, first-principle calculations suggest that Cu dopants in CdTe can occupy the Cd atomic site acting as an acceptor, as well as the interstitial positions acting as a donor [20] . Originally, Cu has been added to the back contact of CdTe solar cells with the purpose of improving the contact properties of CdTe by forming a degenerate semiconductor layer, for example, in the form of Cu x Te, Cu-doped ZnTe, HgTe:CuTe-doped graphite paste or As 2 Te 3 :Cu [5] , [21] , [22] , [23] , [24] . During back contact processing, part of the Cu has also been found to diffuse into CdTe [25] , [26] , where it increases acceptor concentration and affects carrier lifetime. In substrate configuration Cu is commonly added to the devices using the same approach as developed for devices in superstrate configuration, that is, the use of a Cu-containing layer with an equivalent Cu thickness of several nanometres in the electrical back contact structure [15] , [16] , [18] . However, this approach is not suitable, because high-temperature steps during subsequent device fabrication lead to excessive diffusion of the mobile Cu into the adjacent layers, deteriorating their electronic properties. This results in drastic performance degradation of the devices and low reproducibility. Attempts have also been made to apply Cu at different processing steps by dipping the cell into warm CuCl solution; however, efficiencies remained ~7% (ref. 27 ). Previously presented approaches did not prove suitable to achieve desired bulk doping of the CdTe layer in substrate configuration, and hence the cell efficiencies remained very low. In this work, the controlled Cu doping of the CdTe layer is achieved by vapour deposition of Cu and subsequent annealing. A small amount of Cu with the equivalent thickness of less than a monolayer is deposited on top of the recrystallized CdTe and diffusion into CdTe is promoted by annealing at 400 °C. This has enabled us to produce CdTe solar cells in substrate configuration with unprecedented high efficiencies. Cu doping of CdTe thin films We have investigated the effect of Cu doping on the resistivity of CdTe layers on glass after CdCl 2 treatment ( Fig. 2a ). Adding 0.8 × 10 15 Cu atoms per cm 2 (sub-monolayer with equivalent thickness of 1 Å) to a 5μm thick CdTe layer results in an abrupt decrease in resistivity by three orders of magnitude and an increase in hole density from <10 12 cm −3 to 3.8 (±0.6) × 10 14 cm −3 as determined by Hall effect measurements. Addition of more Cu leads to a small increase in CdTe resistivity accompanied by a decrease in hole density (2.8 (±0.1) × 10 13 cm −3 for addition of 8 × 10 15 Cu atoms per cm 2 ) owing to the formation of compensating donor-type defects. This demonstrates that the hole density in polycrystalline CdTe can be maximized by carefully controlling the concentration of the dopant. 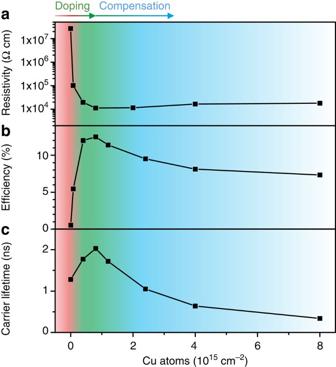Figure 2: Influence of Cu doping on electrical properties of CdTe thin films and solar cells. (a) Resistivity measurements of CdCl2treated CdTe thin films on glass doped with different amounts of Cu. The regions of doping and compensation are indicated by the colour shading. (b) Efficiency of CdTe solar cells in substrate configuration doped with different amounts of Cu. (c) Minority carrier lifetime in the CdTe layer of completed solar cells as determined by TRPL measurements. Figure 2: Influence of Cu doping on electrical properties of CdTe thin films and solar cells. ( a ) Resistivity measurements of CdCl 2 treated CdTe thin films on glass doped with different amounts of Cu. The regions of doping and compensation are indicated by the colour shading. ( b ) Efficiency of CdTe solar cells in substrate configuration doped with different amounts of Cu. ( c ) Minority carrier lifetime in the CdTe layer of completed solar cells as determined by TRPL measurements. Full size image Cu doping of CdTe solar cells We have investigated Cu distribution in CdTe solar cells in substrate configuration with a 5μm thick absorber and 1.0 × 10 15 Cu atoms per cm 2 by secondary ion mass spectroscopy (SIMS) measurements ( Fig. 3 ). Accumulation of Cu at the CdTe/back contact interface and in the n-type CdS is observed. The Cu concentration in the polycrystalline CdTe is 5 (±3) × 10 17 cm −3 (see Methods), in agreement with measurements of devices in superstrate configuration [28] . 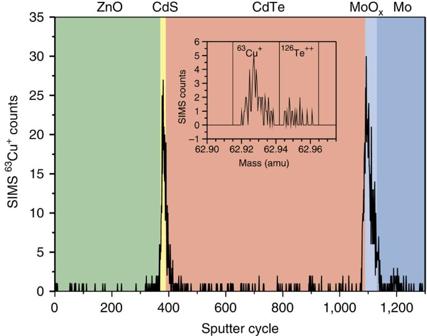Figure 3: Distribution of Cu in a completed solar cell. SIMS measurement of the depth dependant Cu distribution in a completed solar cell doped with Cu using 1.0·1015Cu atoms per cm2deposited on the CdTe layer. Cu preferentially accumulates at the CdTe/back contact interface and in the CdS. The inset shows the mass spectrum around the mass of63Cu+in the CdTe layer from sputter cycle 500 to 1,000. Cu is present in the CdTe layer and the mass of63Cu+is distinguishable from126Te++. Figure 3: Distribution of Cu in a completed solar cell. SIMS measurement of the depth dependant Cu distribution in a completed solar cell doped with Cu using 1.0·10 15 Cu atoms per cm 2 deposited on the CdTe layer. Cu preferentially accumulates at the CdTe/back contact interface and in the CdS. The inset shows the mass spectrum around the mass of 63 Cu + in the CdTe layer from sputter cycle 500 to 1,000. Cu is present in the CdTe layer and the mass of 63 Cu + is distinguishable from 126 Te ++ . Full size image To study the depth-dependent collection efficiency of the solar cells, we have performed electron beam-induced current (EBIC) measurements ( Fig. 4a,b ). In a Cu-free cell, the only carriers that are efficiently collected are those that are generated close to the electrical back contact. Upon optimum Cu doping, the effective carrier collection is observed in a region close to the CdS. Effective carrier collection is desirable in a region where carriers are generated by the incoming sunlight. Over 90% of the usable sunlight is absorbed in the first micrometre of the CdTe layer near the interface to the n-type CdS layer. As such, Cu doping shifts the region of effective carrier collection to the region of carrier generation, resulting in a dramatic increase in efficiency from <1% to >12% ( Fig. 2b ). All solar cell parameters are improved and the quantum efficiency (QE) increases from ~10% to ~90% ( Fig. 5a,b ). The QE of the Cu-free cell exhibits highest values for photons with wavelength of 800–850 nm, which have a higher probability of penetrating deeper into the CdTe layer towards the region of effective carrier collection. 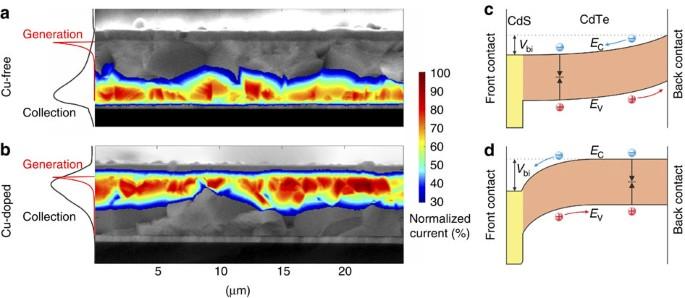Figure 4: EBIC measurements and energy band diagrams. (a,b) EBIC measurements of CdTe solar cells processed without Cu (a) and with 1 × 1015Cu atoms per cm2(b). The Cu-doped cell collects current at the front side of the solar cell, whereas the Cu-free cell collects current more efficiently at the back side. EBIC signal was normalized to 100%. For better visualization, EBIC signal <30% is not shown. Grain contrast arises from topography due to cleaving of the sample. The profiles on the left show the horizontally averaged EBIC signal (black, collection). Furthermore, a schematic of the depth-dependent carrier generation under normal operation in sunlight is shown (red, generation). (c,d) Proposed energy band diagrams for CdTe solar cells without (c) and with optimum Cu doping (d). The Cu-free cell has a small band bending and small electric field close to the CdS. Therefore, electron-hole pairs have a high probability to recombine before they are collected. Only close to the electrical back contact, energy bands are sufficiently bent and carriers are collected. Energy bands of the Cu-doped cell are bent close to the CdS/CdTe junction, leading to efficient carrier collection close to the CdS. Conduction band energyEC, valence band energyEVand built-in voltageVbiare indicated. Figure 4: EBIC measurements and energy band diagrams. ( a , b ) EBIC measurements of CdTe solar cells processed without Cu ( a ) and with 1 × 10 15 Cu atoms per cm 2 ( b ). The Cu-doped cell collects current at the front side of the solar cell, whereas the Cu-free cell collects current more efficiently at the back side. EBIC signal was normalized to 100%. For better visualization, EBIC signal <30% is not shown. Grain contrast arises from topography due to cleaving of the sample. The profiles on the left show the horizontally averaged EBIC signal (black, collection). Furthermore, a schematic of the depth-dependent carrier generation under normal operation in sunlight is shown (red, generation). ( c , d ) Proposed energy band diagrams for CdTe solar cells without ( c ) and with optimum Cu doping ( d ). The Cu-free cell has a small band bending and small electric field close to the CdS. Therefore, electron-hole pairs have a high probability to recombine before they are collected. Only close to the electrical back contact, energy bands are sufficiently bent and carriers are collected. Energy bands of the Cu-doped cell are bent close to the CdS/CdTe junction, leading to efficient carrier collection close to the CdS. Conduction band energy E C , valence band energy E V and built-in voltage V bi are indicated. 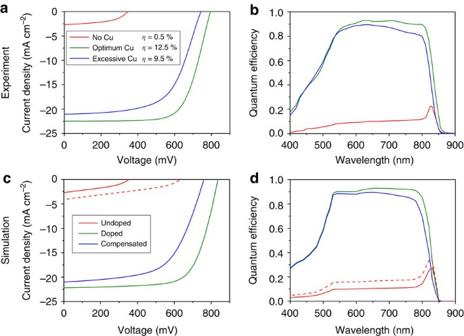Figure 5:J–Vand QE curves of CdTe solar cells doped with different amounts of Cu. (a,b)J–V(a) and QE (b) measurements of CdTe solar cells processed without Cu, with optimum Cu (8 × 1014Cu atoms per cm2) and with excessive Cu (2.4 × 1015Cu atoms per cm2). Efficiencies (η) of the corresponding cells are given in the inset. (c,d) Simulations ofJ–V(c) and QE (d) characteristics of CdTe solar cells with undoped (no acceptors), doped (6.5 × 1014cm−3acceptors) and compensated (1 × 1015cm−3acceptors and 0.9 × 1015cm−3donors) absorber. The undoped sample is simulated both with standard (0.4 eV, dashed line) and with increased (0.7 eV, solid line) valence band energy barrier at the CdTe/back contact interface. Full size image Figure 5: J–V and QE curves of CdTe solar cells doped with different amounts of Cu. ( a , b ) J–V ( a ) and QE ( b ) measurements of CdTe solar cells processed without Cu, with optimum Cu (8 × 10 14 Cu atoms per cm 2 ) and with excessive Cu (2.4 × 10 15 Cu atoms per cm 2 ). Efficiencies ( η ) of the corresponding cells are given in the inset. ( c , d ) Simulations of J–V ( c ) and QE ( d ) characteristics of CdTe solar cells with undoped (no acceptors), doped (6.5 × 10 14 cm −3 acceptors) and compensated (1 × 10 15 cm −3 acceptors and 0.9 × 10 15 cm −3 donors) absorber. The undoped sample is simulated both with standard (0.4 eV, dashed line) and with increased (0.7 eV, solid line) valence band energy barrier at the CdTe/back contact interface. Full size image We have used the 1D simulation software SCAPS [29] to investigate the influence of doping on current density–voltage ( J–V ) and QE curves ( Fig. 5c,d ). QE simulation of a solar cell without acceptor doping of the absorber confirms the experimentally obtained curve for the cell without Cu addition. For the simulation of the Cu-doped device, acceptor-type defects with a concentration of 6.5 × 10 14 cm −3 were introduced into CdTe in order to obtain a hole density of 3.8 × 10 14 cm −3 consistent with Hall effect measurements. This results in a change in the QE as observed upon Cu addition. To reproduce the observed behaviour of the open-circuit voltage ( V OC ) completely, the valence band energy barrier at the CdTe/back contact interface is increased in the simulation of the sample without acceptor doping. Cu reduces this barrier [21] , [30] and accumulates at the CdTe/back contact interface as observed with SIMS measurements ( Fig. 3 ). Excessive Cu doping leads to a decrease of all solar cell parameters and a reduced QE in the long wavelength region ( Fig. 5a,b ). The net hole density is reduced and the minority carrier lifetime decreases, as confirmed with time-resolved photoluminescence (TRPL) measurements ( Fig. 2c ). In simulations, an increase of the acceptor-type defect concentration to 1 × 10 15 cm −3 together with the introduction of compensating donor-type defects with a concentration of 9 × 10 14 cm −3 reproduce J–V and QE curves of the sample with excess Cu ( Fig. 5c,d ). The results support an explanation of the reduced device performance with excessive Cu doping by the formation of deep donors, which act as recombination centres. Record efficiency solar cells The controlled doping of CdTe has enabled the achievement of efficiencies up to 13.6% for CdTe solar cells in substrate configuration on glass substrates ( Fig. 6 and Table 1 ). The open-circuit voltage ( V OC =852 mV) and fill factor (FF=75.3%) are especially noteworthy as they almost reach the values of record efficiency cells in superstrate configuration ( V OC =857 mV, FF=79.0% (ref. 31 and Green M.A., personal communication)), whereas earlier substrate configuration devices have especially suffered from low FF values, mostly <60% (refs 14 , 17 ). This proves for the first time that the CdS/CdTe junction and electrical back contact of devices in substrate configuration can be produced with a quality comparable to the record superstrate device. The QE measurement ( Fig. 6b ) shows the potential for further efficiency improvement by reducing CdS layer thickness in order to increase the short-circuit current density ( J SC ) and to close the efficiency gap to superstrate configuration. The reduction of CdS thickness will require further optimization work, similar to what has been done for CdTe solar cells in superstrate configuration [32] . 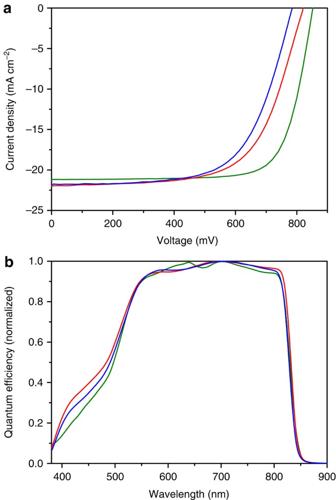Figure 6:J–Vand QE measurements of CdTe solar cells. (a)J–Vmeasurements of CdTe solar cells in substrate configuration on glass (green), molybdenum foil (red), and steel foil (blue) substrates. The corresponding PV parameters and efficiency are given inTable 1(Samples A, E, and F). (b) QE measurements of the corresponding cells. The loss in the QE for wavelengths below ~550 nm is caused by the absorption in the CdS layer, showing the large potential for further improvement inJSCand efficiency by reducing the CdS layer thickness. Figure 6: J–V and QE measurements of CdTe solar cells. ( a ) J–V measurements of CdTe solar cells in substrate configuration on glass (green), molybdenum foil (red), and steel foil (blue) substrates. The corresponding PV parameters and efficiency are given in Table 1 (Samples A, E, and F). ( b ) QE measurements of the corresponding cells. The loss in the QE for wavelengths below ~550 nm is caused by the absorption in the CdS layer, showing the large potential for further improvement in J SC and efficiency by reducing the CdS layer thickness. Full size image Table 1 Photovoltaic parameters of selected CdTe solar cells. Full size table Several samples with efficiencies of >13% were produced and Table 1 shows the photovoltaic parameters of a selection of cells, demonstrating the good reproducibility of the process. As a proof of concept, we have applied the process on metal foils and have achieved efficiencies of 11.5% and 10.9% on molybdenum and steel foil substrates, respectively ( Fig. 6 and Table 1 ). This greatly exceeds the previous record efficiency of 7.8% (ref. 13 ), proving that highly efficient flexible CdTe solar cells on non-transparent substrates are possible. We expect to close the remaining gap between efficiencies on glass and on metal foil substrates by adapting processing temperatures to the changed thermal mass of the substrate and by reducing impurity diffusion from the steel foil substrate through the application of improved diffusion barrier layers. The possibility of high deposition rates of CdTe with a simple evaporation process—benefiting from the congruent evaporation characteristics—offers low-cost high-speed processing advantages for flexible CdTe solar cells whereas complex multinary compounds, such as Cu(In,Ga)Se 2 absorbers, require sophisticated composition control for high-efficiency solar cells. Furthermore, the superior temperature coefficient of CdTe photovoltaics compared to Si wafers and Cu(In,Ga)Se 2 is advantageous during field operation, especially in hot climates [33] . Cu is known to influence stability of CdTe solar cells [23] , [24] , [34] , [35] . It was found that excess Cu at the back contact reduces device stability as it can diffuse towards the junction [23] , [35] . In the case of the presented Cu doping method, a controlled amount of Cu is added close to the front contact. This approach is expected to avoid excessive Cu diffusion from the back contact towards the junction, which could translate to improved device stability. After storage of the record efficiency sample at room temperature under indoor illumination for more than 6 months, the efficiency of the best cells was unchanged at 13.6%, indicating good stability of the cells. Standardized stability tests of encapsulated cells for long durations are the subject of further investigations. The results show that the electronic properties of CdTe and the efficiency of the solar cells can be enhanced by carefully controlling Cu doping of the CdTe. These observations can be explained by the amphoteric doping behaviour of Cu in CdTe. Cu addition up to an optimum amount increases acceptor concentration, for example, due to the formation of Cu Cd . Further increase in Cu concentration decreases hole density and carrier lifetime owing to the formation of compensating donor-type defects, for example, copper interstitials [20] . The Cu concentration in the doped polycrystalline CdTe is three orders of magnitude higher than the measured hole density of 3.8 × 10 14 cm −3 . Part of the difference is attributed to the fact that the Cu Cd acceptor has a large activation energy. However, according to numerical simulations only 6.5 × 10 14 Cu atoms per cm 3 are required to obtain the measured hole density (see Methods). The main part of the difference between the measured Cu concentration and hole density is attributed to the preferential accumulation of Cu at grain boundaries, which is energetically favored [36] . Cu doping changes the position of effective carrier collection as measured with EBIC. This is explained with the energy band diagrams in Fig. 4c,d . A Cu-free cell has a space charge region (SCR) that extends over the whole ~5μm absorber as confirmed with capacitance–voltage ( C–V ) measurements. The low acceptor concentration leads to a small electric field—the result being that carriers are collected less efficiently even in the SCR. Only close to the electrical back contact, Fermi level pinning at the CdTe/back contact interface can cause sufficient band bending to allow efficient collection of carriers. Doping CdTe with 1 × 10 15 Cu atoms per cm 2 results in a SCR of ~1.8 μm (from C–V measurements) and causes sufficient band bending close to the CdS to generate a strong electric field, leading to effective carrier collection ( Fig. 4b ). We found that substrate and superstrate configuration solar cells need different Cu addition methods to achieve good electronic properties. Comparison of the resulting Cu distributions [28] ( Fig. 3 ) shows that both methods lead to accumulation of Cu at the CdTe/back contact interface and in the CdS as well as a small Cu concentration in the CdTe. The amount of Cu at the electrical back contact strongly differs in the two configurations, whereas the Cu concentration in the CdTe layer is similar, supporting the importance of the precise control of Cu concentration in the CdTe layer in order to maximize its hole density. To conclude, we have introduced an innovative concept for the development of CdTe solar cells in substrate configuration, which enables efficiencies of 13.6% and 11.5% on glass and on metal foil substrates, respectively, demonstrating the feasibility to obtain highly efficient CdTe solar cells on flexible metal foil substrates. This is achieved by precisely controlled Cu doping of CdTe resulting in reduced compensation of acceptors, increased hole density, optimized carrier lifetime and a pronounced improvement of the collection of photo-generated charge carriers in CdTe close to the CdS/CdTe junction. The results offer new opportunities in CdTe PV research to increase V OC towards 1 V through further improved doping procedures. Substrate configuration growth allows better control of p-type doping of the absorber in the absence of the n-type CdS layer and decouples doping processes from the junction formation, which is a significant advantage over superstrate configuration [37] . Finally, the results not only open up new research directions but also pave the way for the industrialization of very cost-efficient solar modules. Sample preparation Solar cells were grown on Corning 7059 borosilicate glass, on flexible molybdenum foil (50μm thickness) and on flexible steel foil substrates (30μm thickness). On steel foil, a Ti/TiN impurity diffusion barrier layer with a thickness of 60/230 nm was deposited by pulsed DC sputtering. On all samples, a 600nm thick Mo electrical back contact layer was deposited by DC sputtering followed by vacuum evaporation of 150 nm of MoO 3 (Alfa Aesar, 99.9995%) and 50 nm of Te layers (Alfa Aesar, 99.9999%). CdTe (5 N Plus Inc., 99.9999%) with a thickness of 4–6μm was deposited by high vacuum evaporation at a substrate temperature of 350 °C followed by deposition of 400 nm of CdCl 2 (Aldrich, 99.995%) and annealing at 435 °C in an oxygen-containing ambient. Cu was deposited by high-vacuum evaporation and diffusion of Cu into CdTe was promoted by annealing at 400 °C in an oxygen-containing ambient. CdS was grown using chemical bath deposition with a thickness of 50–100 nm, followed by a CdCl 2 treatment. Another CdS layer was subsequently deposited as before. A bilayer front contact of i-ZnO and ZnO:Al was prepared by rf-sputtering. A metallic Ni/Al grid was applied for improved front contact conductivity and 85 nm of MgF 2 was deposited as anti-reflection coating. The cell area was defined by mechanical scribing. The completed solar cells were annealed at 190–250 °C. The evaporated Cu layer had an equivalent thickness of between 0.1 and 10 Å, which corresponds to 8 × 10 13 and 8 × 10 15 Cu atoms per cm 2 . Cu was evaporated at a rate of 0.03 Å s −1 and the Cu thickness was controlled with a quartz crystal microbalance, which was calibrated by evaporating 50 nm of Cu on a glass slide at a rate of 0.03 Å s −1 and measuring the resulting thickness with a profilometer. Samples for CdTe resistivity and Hall effect measurements were prepared by depositing CdTe layers with a thickness of 5 μm on Corning 7059 borosilicate glass followed by a CdCl 2 treatment and Cu doping as described above. The electrical contacts were made by vacuum evaporation of Au through a mask. For resistivity measurements, line contacts with different distances between 0.2 and 2 mm were used, and for Hall effect measurements, point contacts in van der Pauw geometry were employed. Resistivity measurements In-plane resistivity of CdTe thin films was measured at room temperature in the dark using a Keithley 2400 Source Meter. The contact resistance was separated from bulk resistance using the transmission-line method by altering the contact distance from 0.2 mm to 2 mm. The contact resistance was found to be <7% of the total resistance at 2mm contact distance. Hall effect measurements Hall effect measurements of CdTe thin films were performed with a HMS 3000 Hall effect measurement system at room temperature in the dark using van der Pauw geometry. The given error is the s.d. of the mean of >10 measurements. Secondary ion mass spectroscopy Cu distribution in the solar cell was measured with a TOF-SIMS [5] from ION-TOF using dual beam depth profiling. Bi 1 + ions with an energy of 25 keV and a current of 1 pA were used as primary ions. An area of (100 μm) 2 was analysed and positive secondary ions were detected. Sputtering of an area of (300 μm) 2 was performed using O 2 + at an energy of 2 kV and a current of 400 nA. The SIMS Cu counts in CdTe were quantified by comparing the normalized Cu SIMS signal ( 63 Cu + / 114 Cd + ) in the absorber with the normalized Cu SIMS signal of a CdTe thin film on Mo/glass with a known Cu concentration. The Cu concentration in the CdTe thin film was determined using inductively coupled plasma mass spectrometry. Inductively coupled plasma mass spectrometry For quantification of Cu traces in Cu-doped CdCl 2 -treated CdTe thin films on Mo/glass, an Agilent 7500ce ICPMS apparatus was used, performing external calibration from certified single elemental standards (1 mg ml −1 ). Only high-purity PE-LD or Teflon vessels were employed during sample preparation and measurement. For the analysis, ~25 mg of the absorber was scratched with the tip of a glass pasteur pipette from the Mo layer and dissolved in 10 ml 65% nitric acid. Afterwards, the acidic solution was adjusted to a final volume of 50 ml with deionized water. For quality assurance, a reference material (NIST SRM 1643e) and spiking of known Cu concentrations to the measurement solution was conducted, resulting in recoveries not lower than 90%. Electron beam-induced current EBIC measurements were performed in a FEI Strata 235 Dual Beam focused ion beam and secondary electron microscopy at accelerating voltage of 25 keV without applied bias at the cell. The current was measured with a SR570 Preamplifier from SRS at a gain of 10 7 . Samples were prepared by mechanical cleaving and electrical contacts to the front and back contact were made with silver paste and indium wires. C–V measurements C–V measurements of solar cells were performed at 30 °C with a frequency of 3 × 10 5 Hz, an oscillating voltage of 50 mV, and bias voltages between −1.5 and +0.5 V. The capacitance was measured with an Agilent E4980A precision LCR meter. The SCR width d SCR at 0 V bias of a solar cell with area A was calculated assuming a plate capacitor with capacitance C =ε 0 ε r A / d SCR , with the vacuum permittivity ε 0 , and a relative dielectric constant ε r =10. Time-resolved photoluminescence TRPL was used to measure minority carrier lifetime in the CdTe layer of the solar cells. TRPL was measured with a near infrared compact fluorescence lifetime spectrometer C12132 by Hamamatsu using a YAG excitation laser with a wavelength of 532 nm, an excitation power of 42.4 mW and a repetition rate of 15 kHz. A high laser power was chosen to characterize the recombination properties in CdTe in the presence of a junction [38] . The detection wavelength was set to the photoluminescence maximum at 825 nm and light was detected using a photomultiplier tube. The lifetime was evaluated using deconvolution and fitting of the initial section of the PL decay with a single exponential function [39] . Solar cell performance measurements J–V characteristics of solar cells were measured under simulated standard-test conditions (25 °C, 1,000 W m −2 , AM 1.5 G illumination) in a sun-simulator. The spectral mismatch correction was performed using QE measurements. The QE of the solar cells was measured with a lock-in amplifier. A chopped white light source (900 W, halogen lamp, 360 Hz) and a dual grating monochromator generated the probing beam. A certified mono-crystalline Si cell from Fraunhofer ISE was used as the reference cell. Cell temperature was controlled at 25 °C with peltier cooling and white light bias was applied. J–V and QE characteristics of the CdTe solar cells on molybdenum and steel foil substrates were independently measured and certified by Fraunhofer ISE, Freiburg, Germany. Simulations The 1D solar cell simulation software SCAPS (version 3.1.02) was used for simulations of J–V and QE measurements [29] . The SCAPS definition file CdTe-base.def (22.5.2009) was used for simulation of the optimally doped sample with the following modifications: CdTe and CdS layer thicknesses were set to 5 μm and 100 nm, ZnO electron affinity was set to 4.4 eV instead of using the value of SnO x , and hole capture cross-section of the donor-type mid-gap defect in CdTe was set to 1 × 10 −13 cm 2 . A series resistance of 3Ω cm 2 was included and reflection was reduced to 6%. To simulate the relatively deep acceptor-type defect states of Cu in CdTe, the shallow acceptor concentration in CdTe was set to zero and an acceptor-type defect with energy of 220 meV above the valence band (Cu Cd ) (ref. 20 ) was introduced. Acceptor-type defect concentration was set to 6.5 × 10 14 cm −3 and hole and electron cross-sections of 1 × 10 −15 cm 2 were used. The concentration was chosen to obtain a hole density of 3.8 × 10 14 cm −3 in the CdTe layer outside the SCR consistent with the value determined by Hall effect measurements. The cell without Cu doping was simulated by using the aforementioned values with the concentration of the acceptor-type defect set to zero. Furthermore, the majority carrier barrier height at the electrical back contact was set to 0.7 eV instead of the default value of 0.4 eV. For simulation of the sample with excessive Cu doping, the aforementioned values of the optimally doped sample were used but the concentration of the acceptor-type defect was increased to 1 × 10 15 cm −3 . Furthermore, a compensating donor-type defect was introduced with a concentration of 9 × 10 14 cm −3 , energy of 380 meV below the conduction band (Cu i ) (ref. 20 ), and electron and hole capture cross-sections of 1 × 10 −11 cm 2 and 2 × 10 −14 cm 2 , respectively. The energetic position of the acceptor-type defect Cu Cd is under debate. Proposed values range between 150 and 350 meV above the valence band. The value from Wei et al . [20] of 220 meV is used for the simulations. How to cite this article: Kranz, L. et al . Doping of polycrystalline CdTe for high-efficiency solar cells on flexible metal foil. Nat. Commun. 4:2306 doi: 10.1038/ncomms3306 (2013).